Cyclic electron flow is redox-controlled but independent of state transition Photosynthesis is the biological process that feeds the biosphere with reduced carbon. The assimilation of CO 2 requires the fine tuning of two co-existing functional modes: linear electron flow, which provides NADPH and ATP, and cyclic electron flow, which only sustains ATP synthesis. Although the importance of this fine tuning is appreciated, its mechanism remains equivocal. Here we show that cyclic electron flow as well as formation of supercomplexes, thought to contribute to the enhancement of cyclic electron flow, are promoted in reducing conditions with no correlation with the reorganization of the thylakoid membranes associated with the migration of antenna proteins towards Photosystems I or II, a process known as state transition. We show that cyclic electron flow is tuned by the redox power and this provides a mechanistic model applying to the entire green lineage including the vast majority of the cases in which state transition only involves a moderate fraction of the antenna. The injection of energy into the biosphere relies on photosynthesis. Solar energy is transiently stored in the form of carbohydrates ensuing from the assimilation of carbon dioxide by the Benson–Calvin cycle [1] . To turnover, this metabolic cycle demands its substrates, ATP and NADPH, to be delivered in a strict stoichiometry of 3/2. It is commonly accepted that, to comply with this requirement, the photosynthetic electron transfer operates according to two different modes, linear (LEF) and cyclic electron flow (CEF), both being indispensable [2] , [3] , [4] . While the former provides ATP and NADPH in a 2.6/2 ratio, the latter exclusively drives phosphorylation [5] and thus supplies the remaining ATP. The fine tuning of these two modes is thus vital, in essence, but its mechanism remains poorly understood. In this context, the fact that the photosynthetic electron chain may undergo another massive reorganization owing to state transitions (ST) has provided a tempting and simple model for the switch between LEF and CEF [6] , [7] , [8] , [9] . ST consists in the lateral migration of the mobile Light Harvesting Complex II (LHCII) from (to) the Photosystem (PS) II-containing stacked regions of the thylakoid to (from) the Photosystem (PS) I-containing stroma lamellae, thereby balancing the excitonic flux between the two photosystems [10] . In the unicellular green alga Chlamydomonas reinhardtii , this lateral redistribution may involve up to 80% of the antenna [11] , and several functional studies supported the tight correlation between this structural rearrangement and the promotion of CEF as illustrated in Fig. 1 (refs 8 , 12 ) . This model reached its acme with the isolation—from Chlamydomona s cells placed in a state denoted as State 2 that promotes the association of the mobile LHCII to PS I—of a super-complex associating PSI and cytochrome b 6 f , driving CEF in vitro [13] , [14] . This finding provided an answer at the molecular level to the question as to how the same individual blocks within an electron transfer chain can contribute to two completely different functional modes. Despite this achievement, what truly governs the formation of these supercomplexes and the promotion of CEF remains equivocal: are they brought about by the kinase-controlled transition to State 2 that drives lateral redistribution of a mobile phosphorylated antenna, or are they an independent effect of the strongly reducing conditions used to trigger state transitions? 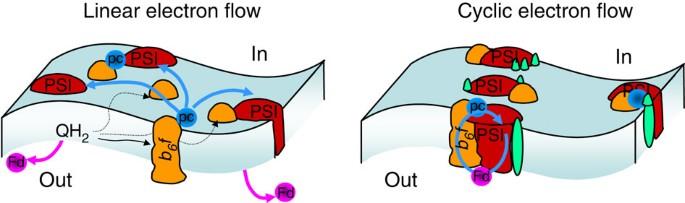Figure 1: A schematic picture of the linear and cyclic electron flow. Cytochromeb6f, PS I, plastocyanin and ferredoxin are respectively depicted in orange, red, blue and purple. In linear electron flow (LEF), shown on the left, the different components of the chain are independent entities and the mobile electron carriers, quinones, plastocyanin and ferredoxin, freely shuttle electrons between the membrane-bound complexes and to FNR. On the contrary, in the cyclic electron flow (CEF) mode, supercomplexes are formed, which comprise, among others, cytochromeb6fand PS I. The formation of these supramolecular edifices is thought to involve the association of the mobile LHCII proteins depicted in green. Figure 1: A schematic picture of the linear and cyclic electron flow. Cytochrome b 6 f , PS I, plastocyanin and ferredoxin are respectively depicted in orange, red, blue and purple. In linear electron flow (LEF), shown on the left, the different components of the chain are independent entities and the mobile electron carriers, quinones, plastocyanin and ferredoxin, freely shuttle electrons between the membrane-bound complexes and to FNR. On the contrary, in the cyclic electron flow (CEF) mode, supercomplexes are formed, which comprise, among others, cytochrome b 6 f and PS I. The formation of these supramolecular edifices is thought to involve the association of the mobile LHCII proteins depicted in green. Full size image By using mutants of C. reinhardtii locked in States 1 or 2 irrespective of the ambient redox conditions, we show that CEF rates as well as formation of CEF supercomplexes that are thought to contribute to the enhancement of CEF, are promoted in reducing conditions with no correlation with ST. Decoupling state transition from the redox poise We recently identified a C. reinhardtii mutant lacking Ptox2 (ref. 15 ), the plastid oxidase that controls the redox state of the plastoquinol pool in the dark [16] . This deficiency results in the plastoquinone pool being predominantly reduced in the dark even in aerobic conditions [15] , so that, in contrast to the wild type, this mutant is in State 2 when the culture is well aerated in the dark, the mobile LHC II being associated with PS I. This is further illustrated in Fig. 2a that compares the phosphorylation pattern of the wild-type, ptox2 and stt7 strains. The latter strain is locked in State 1 because of the absence of the Stt7 kinase, which is responsible for phosphorylation of the mobile antenna in State 2, upon reduction of the plastoquinone pool [17] , [18] , [19] . We compared three different conditions expected to promote, to a different extent, States 1 or 2. The archetypical State 1 was obtained in oxic conditions, with light and inhibition of PS II by addition of 3-(3,4-dichlorophenyl)-1,1-dimethylurea (DCMU) promoting complete oxidation of the plastoquinone pool [20] , [21] . The wild type displayed a phosphorylation pattern identical to that observed with stt7 —a reference for State 1—with no detectable phosphorylation of the LHCII proteins P13 and P17 and low levels of phosphorylation of P11, CP26 and CP29 (refer to Minagawa and Takahashi [22] and Minagawa [23] for the correspondence between proteins and lhcb gene nomenclature). A similar State 1-type phosphorylation pattern was observed with the ptox2 mutant kept under illumination in the presence of DCMU, albeit slightly less pronounced than in the wild type or stt7 cases. In anoxic conditions, sst7 cells retained a phosphorylation pattern typical of State 1, despite some limited increase in the phosphorylation of P11, CP29 and CP26 subunits, as previously reported [18] , [19] , whereas the wild type and ptox2 strains displayed similar phosphorylation patterns typical of State 2, with a high phosphorylation level of P11, CP29 and CP26 (refs 17 , 18 , 19 ) [17] , [18] , [19] and a significant phosphorylation of the LHCII proteins P13 and P17. When kept in oxic conditions under vigorous stirring in the dark, the phosphorylation pattern of ptox2 remained typical of State 2, being almost identical to that obtained in anoxic conditions. In contrast, proper aeration of the wild type, by vigorous stirring in the dark, established a quasi-State 1 situation as previously reported [24] . From a functional stand-point, the main consequence of the antenna phosphorylation is that it promotes their lateral migration and their association to PSI. This can be probed by measuring the relative PS II and PSI antenna size via low-temperature emission spectra. Consistent with the phosphorylation patterns, ptox2 and the wild type displayed similar spectra as stt7 when State 1 was promoted with light and DCMU ( Fig. 2b , central panel). However, as shown in Fig. 2b (left panel), the spectrum obtained with the wild type aerated in darkness was almost identical to that of stt7 cells and was characteristic of State 1, whereas for ptox2 , as previously reported [15] , the long wavelength emitting components prevailed in both oxic (dark and vigorous stirring) and anoxic conditions, showing excitonic coupling of the mobile antennae to PS I ( Fig. 2b , left and right panels). 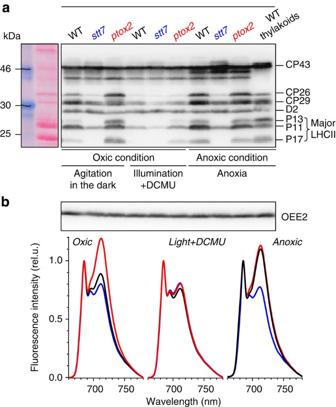Figure 2: Characterization of the three strains used in this study. Panelashows an immunoblot with an anti-phosphothreonine antibody of wild type,stt7andptox2cells in two oxic conditions and in anoxia. When illuminated in the presence of DCMU (center), all strains displayed a similar pattern, typical of State 1, with little -if any- phosphorylation of P13 and P17 and low phosphorylation of P11, CP26 and CP29. In anoxic conditions (right), the wild type andptox2- but notstt7-, showed a marked increase in phosphorylation of P11, P13, P17, CP29 and CP26, in good agreement with (refs17,19). In thestt7strain, the phosphorylation level of P17 and P13 remained unchanged despite a small increase in P11, CP26 and CP29 phosphorylation as reported in the study by Lemeilleet al.19When stirred in the dark (left),ptox2cells showed a pattern similar to the anoxic condition, indicating State 2, in contrast tostt7cells, which were similar to the light+DCMU condition (State1). In these conditions, the wild type also showed a pattern similar to State 1, albeit with a low level of P13 and P17 phosphorylation indicating low level activation of the kinase. OEE2 was used as a loading control. Panelbshows the low-temperature emission spectra, diagnostic of the relative absorption cross section of PS I and II. The spectra have been normalized to their amplitude at 685 nm. Two mains peaks are resolved at 684 nm and in the 715 nm region, which respectively correspond to fluorescence by PS II and PSI. In the wild type (black spectra), the former is larger than the latter in State 1 (oxic and vigorous stirring in the dark) conditions andvice versain State 2 (anoxic) conditions21. Instt7(blue spectra), light-emission from PS II largely prevailed in both conditions as previously reported17, whereas in theptox2strain (red spectra) light emission was dominated by PSI fluorescence in agreement with the study by Houille-Verneset al.15 Figure 2: Characterization of the three strains used in this study. Panel a shows an immunoblot with an anti-phosphothreonine antibody of wild type, stt7 and ptox2 cells in two oxic conditions and in anoxia. When illuminated in the presence of DCMU (center), all strains displayed a similar pattern, typical of State 1, with little -if any- phosphorylation of P13 and P17 and low phosphorylation of P11, CP26 and CP29. In anoxic conditions (right), the wild type and ptox2 - but not stt7 -, showed a marked increase in phosphorylation of P11, P13, P17, CP29 and CP26, in good agreement with (refs 17 , 19 ). In the stt7 strain, the phosphorylation level of P17 and P13 remained unchanged despite a small increase in P11, CP26 and CP29 phosphorylation as reported in the study by Lemeille et al . [19] When stirred in the dark (left), ptox2 cells showed a pattern similar to the anoxic condition, indicating State 2, in contrast to stt7 cells, which were similar to the light+DCMU condition (State1). In these conditions, the wild type also showed a pattern similar to State 1, albeit with a low level of P13 and P17 phosphorylation indicating low level activation of the kinase. OEE2 was used as a loading control. Panel b shows the low-temperature emission spectra, diagnostic of the relative absorption cross section of PS I and II. The spectra have been normalized to their amplitude at 685 nm. Two mains peaks are resolved at 684 nm and in the 715 nm region, which respectively correspond to fluorescence by PS II and PSI. In the wild type (black spectra), the former is larger than the latter in State 1 (oxic and vigorous stirring in the dark) conditions and vice versa in State 2 (anoxic) conditions [21] . In stt7 (blue spectra), light-emission from PS II largely prevailed in both conditions as previously reported [17] , whereas in the ptox2 strain (red spectra) light emission was dominated by PSI fluorescence in agreement with the study by Houille-Vernes et al . [15] Full size image This conclusion was further confirmed by the direct measurement of the PS I antenna size. As shown in Fig. 3 for the wild type, for a given light intensity, the rate of ECS build-up upon continuous illumination (for details see Methods) was faster in anoxic than in oxic conditions, reflecting the increased PSI antenna size in State 2. The ratio of anoxic versus oxic charge separation rates was 1.02 and 1.05 in the stt7 and ptox2 strains, versus 1.25, in the wild type ( Table 1 ). Although they do not provide absolute values, these numbers may be discussed in the light of the current knowledge of the number of chlorophyll borne by PS I and II and by the various antenna subunits and the resulting expected extent of antenna size associated with state transition. In C. reinhardtii , each single PSI is connected to nine Lhc-a subunits [25] (versus four in higher plants [26] ) so that the total chlorophyll (Chl) content is ~270 Chl (100 Chl in the core of PSI and 170 distributed among the 9 Lhc-a). Each core PS II bears 35 chlorophylls [27] . Assuming that the two photosystems have the same absorption cross section in State 1, these different Chl contents imply that the peripheral antenna proteins of PS II bear ~235 Chl. This would constitute the pool of Chl connected to PS II in State 1 and susceptible to migrate towards PSI. In C. reinhardtii , the lateral redistribution of the antenna has been reported to involve up to 80% of the PS II mobile antenna [28] , that is, ~180 Chls. If they were connected to PSI, this would yield a 1.5-fold larger antenna, a theoretical value that nicely matches the 1.55 figure experimentally determined in (ref. 29 ). In our experiments, the extent by which the PSI antenna size increased in the wild type was pronounced, but notably smaller (1.27-fold), suggesting that we may predominantly probe in State I, a population of larger antenna size among a heterogeneous PSI population, or that part of the antenna that is disconnected from PS II upon state transition is simply not connected to PSI, as already proposed [30] , [31] , but against the conclusion drawn in the study by Delosme et al . [29] on the absence of disconnected antenna in State 2. In any case, we did observe, as expected, a stark contrast between the wild type and the two other strains, ptox2 or stt7 , in which the transitions from oxic to anoxic conditions hardly affected the PSI absorption cross section (or the 77K fluorescence emission spectrum, see Fig. 2b ). 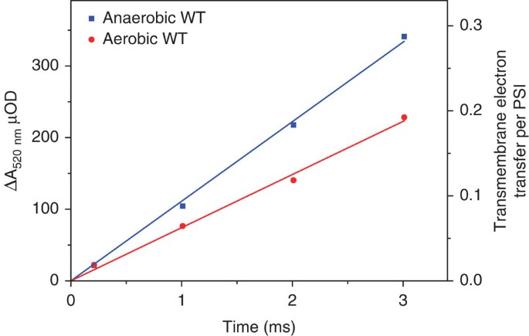Figure 3: Assessing the variation of the PSI antenna size upon ST. The figure shows the time course of the absorption changes measured at 520 nm upon continuous illumination with wild-type cells in oxic and anoxic conditions (after 35 min of anoxia). The rightyaxis was scaled taking as a reference the signal resulting from the transmembrane charge transfer of one electron per PSI, that is, the absorption changes measured upon a single-turnover saturating laser flash in the absence of PS II activity. Figure 3: Assessing the variation of the PSI antenna size upon ST. The figure shows the time course of the absorption changes measured at 520 nm upon continuous illumination with wild-type cells in oxic and anoxic conditions (after 35 min of anoxia). The right y axis was scaled taking as a reference the signal resulting from the transmembrane charge transfer of one electron per PSI, that is, the absorption changes measured upon a single-turnover saturating laser flash in the absence of PS II activity. Full size image Table 1 Photosystem I relative antenna size. Full size table Taking the PSI antenna size of the wild type in oxic (dark and vigorous stirring) as a reference, we found similar figures for wild type and stt7 and a 1.2-fold larger PSI antenna in ptox2 (see Table 1 ). In contrast, we found similar figures in wild type and ptox2 in anoxic conditions that were, respectively, 1.27- and 1.25-fold larger than in stt7 . State II is not sufficient to promote CEF As explained above, the oxic conditions used (dark and vigorous stirring) were appropriate to maintain the association of the mobile antennae to PSI in ptox2 and to PS II in the wild type. Thus, were this association sufficient for an enhanced CEF, the ptox2 mutant would display a more efficient CEF than the wild type in these dark and well aerated, oxic conditions. As depicted in Fig. 4a , this was not the case. CEF was measured through the light-induced redox changes of the chlorophyll dimer of PS I, P 700. In order to inhibit LEF, DCMU was added to the sample just before the measurement as in the study by Alric et al . [32] The steady-state level of photo-induced P 700 + was similar in both strains, and so were the kinetics of reduction of P 700 + in the dark following its full oxidation by a short saturating pulse. After taking into account the different PSI antenna sizes (see Methods section), CEF in the two strains was indistinguishable ( Table 2 ). Thus, State 2 is not sufficient to enhance CEF as previously suggested in the study by Terashima et al . 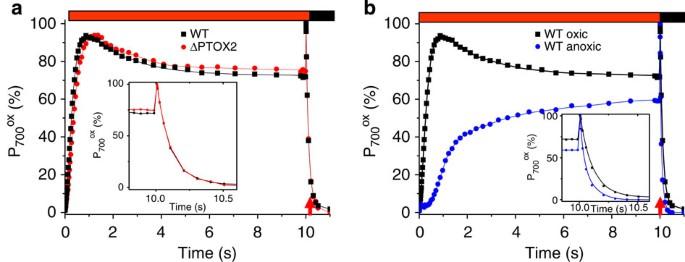Figure 4: Assessing cycling electron flow via the redox changes of P700. As indicated by the red horizontal bar, the samples were submitted to a continuous illumination followed by a pulse of saturating intensity (highlighted by the red arrow). The inset shows a zoom on the reduction of P700+in the dark following this pulse. The left panel shows the redox changes of P700in the wild type andptox2strains in oxic conditions and the right panel compares the kinetics of the redox changes in the wild type in oxic and anoxic conditions. In the former case, the cells were kept in the dark under vigorous stirring to induce State 1 in the wild type and State 2 inptox2 (see text andFig. 2for details). To inhibit LEF and allow the assessment of CEF, DCMU was added just before the measurement. In anoxic conditions, the kinetics were measured after 35 min of incubation in anoxia to alleviate acceptor side limitation. The efficiency of CEF may be assessed via the steady state value of the fraction of P700being reduced (the larger this fraction, the more efficient CEF). [33] Figure 4: Assessing cycling electron flow via the redox changes of P 700 . As indicated by the red horizontal bar, the samples were submitted to a continuous illumination followed by a pulse of saturating intensity (highlighted by the red arrow). The inset shows a zoom on the reduction of P 700 + in the dark following this pulse. The left panel shows the redox changes of P 700 in the wild type and ptox2 strains in oxic conditions and the right panel compares the kinetics of the redox changes in the wild type in oxic and anoxic conditions. In the former case, the cells were kept in the dark under vigorous stirring to induce State 1 in the wild type and State 2 in ptox 2 (see text and Fig. 2 for details). To inhibit LEF and allow the assessment of CEF, DCMU was added just before the measurement. In anoxic conditions, the kinetics were measured after 35 min of incubation in anoxia to alleviate acceptor side limitation. The efficiency of CEF may be assessed via the steady state value of the fraction of P 700 being reduced (the larger this fraction, the more efficient CEF). Full size image Table 2 Cyclic electron transfer rates in the wild type, stt7 and ptox2 strains in oxic and anoxic conditions. Full size table CEF is enhanced in the absence of state transition There must be (an)other parameter(s) that tune(s) the efficiency of CEF to account for its enhancement under the conditions promoting the association of the mobile LHCII to PSI. We thus measured CEF under anoxia, a condition that, owing to the inhibition of mitochondrial respiration and chlororespiration, results in an increase of the intracellular reducing power, and thereby promotes the reduction of the plastoquinone pool which, in turn, triggers the transition to State 2 (ref. 10 ), as shown in Fig. 2 . As illustrated in Fig. 5 , after a few minutes of anoxia, the efficiency of the oxidation of P 700 by light dropped dramatically. This is characteristic of the so-called ‘acceptor side limitation’, whereby reduction of the electron carriers normally acting as electron acceptors promotes the fast charge recombination of the light-induced radical pair [34] , [35] , [36] , [37] . When this occurs, the overall rate of reduction of P 700 + is a combination of electron donation via the cyclic pathway and charge recombination, as depicted in the scheme shown in Fig. 5 , and this precludes a reliable quantification of CEF. Saliently, Fig. 5 also shows that this inhibited situation was only transient. Indeed, after a few tens of minutes of anoxia, the inhibition was entirely alleviated and illumination induced the full oxidation of P 700 . Several hypotheses may account for this relaxation among which the involvement of proteins upregulated in anoxic conditions as reported in the studies by Terashima et al . [33] , [39] and Mus et al . [38] , or simply the onset of fermentation that consumes reducing power to make ATP [6] . We favor the latter hypothesis as 30–40 min were sufficient to relieve the limitation, a time lapse which is shorter than the 2 h required for acclimation due to specific changes in protein expression patterns [33] , [38] , [39] , [40] . In any case, from an experimental stand-point, it allowed the determination of CEF once the acceptor side limitation was alleviated, conditions that, for short, we will hereafter refer to as anoxia. 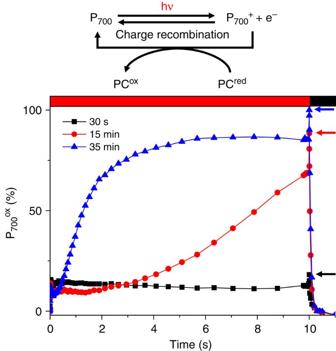Figure 5: The shift from oxic to anoxic conditions results in a transient PSI inhibition. The figure shows the redox changes of the chlorophyll dimer, P700, of PS I. Right after transfer to anoxia, illumination induced hardly any oxidation of P700despite the inhibition of electron donation from PS II by DCMU (10 μM). This indicates the occurrence of a process competing very efficiently with the light-induced oxidation of P700. As depicted in the scheme, the reduction of P700+may involve either the donation of an electron by an external electron donor, here plastocyanin (PC), or charge recombination of the light-induced radical pair. In principle the two pathways co-exist, but the yield of the latter is in general negligible because electron donation from PC is faster than charge recombination. However, when the electron acceptors of PSI are already reduced prior to the light-induced oxidation of P700, the lifetime of the intermediate radical pair, which normally decays quickly owing to the forward electron transfer to these terminal acceptors, is substantially lengthened and this considerably increases the yield of charge recombination. This is why this situation is commonly described as ‘PSI acceptor side limitation’. It can be discriminated from a fast electron donation from the upstream part of the chain by a short pulse of saturating exciting light35. The horizontal arrows indicate the maximum amount for P700that can be oxidized by the pulse in the various conditions. This level was initially ~20% of total photoxidizable P700(measured in oxic conditions), which is diagnostic of a strong acceptor side limitation. However, this situation was transient, as illustrated by the kinetics measured 15 and 35 min after the onset of the anoxia, which showed the progressive restoration of kinetics similar to that of oxic cells. The trace obtained at 35 min was representative of the kinetics measured afterwards. Figure 5: The shift from oxic to anoxic conditions results in a transient PSI inhibition. The figure shows the redox changes of the chlorophyll dimer, P 700 , of PS I. Right after transfer to anoxia, illumination induced hardly any oxidation of P 700 despite the inhibition of electron donation from PS II by DCMU (10 μM). This indicates the occurrence of a process competing very efficiently with the light-induced oxidation of P 700 . As depicted in the scheme, the reduction of P 700 + may involve either the donation of an electron by an external electron donor, here plastocyanin (PC), or charge recombination of the light-induced radical pair. In principle the two pathways co-exist, but the yield of the latter is in general negligible because electron donation from PC is faster than charge recombination. However, when the electron acceptors of PSI are already reduced prior to the light-induced oxidation of P 700 , the lifetime of the intermediate radical pair, which normally decays quickly owing to the forward electron transfer to these terminal acceptors, is substantially lengthened and this considerably increases the yield of charge recombination. This is why this situation is commonly described as ‘PSI acceptor side limitation’. It can be discriminated from a fast electron donation from the upstream part of the chain by a short pulse of saturating exciting light [35] . The horizontal arrows indicate the maximum amount for P 700 that can be oxidized by the pulse in the various conditions. This level was initially ~20% of total photoxidizable P 700 (measured in oxic conditions), which is diagnostic of a strong acceptor side limitation. However, this situation was transient, as illustrated by the kinetics measured 15 and 35 min after the onset of the anoxia, which showed the progressive restoration of kinetics similar to that of oxic cells. The trace obtained at 35 min was representative of the kinetics measured afterwards. Full size image Figure 4b shows that, in the wild-type, the steady-state level of P 700 + was lower in anoxia than in oxic conditions and that its re-reduction in the dark, after its full oxidation by a short saturating pulse, was accelerated. Both observations concur in showing that, in agreement with numerous previous studies [8] , [12] and other studies [41] , [42] , [43] , [44] for discussion, CEF is faster in anoxia. Yet, the nature of the process that governs this enhancement remains to be unraveled. From the experiments with the ptox2 mutant, we concluded that the lateral migration of a mobile LHCII antenna and its binding to PSI are not sufficient for an increased CEF. To understand whether they are, at least, a prerequisite, we measured CEF under anoxia in the stt7 strain. As shown above, its phosphorylation pattern remained typical of State 1 in anoxia, and we observed no significant changes in the PS I absorption cross section upon transition of stt7 from oxic to anoxic conditions ( Fig. 2b and Table 1 ). As indicated in Table 2 , we found no statistically significant differences in CEF between the wild-type and stt7 strains in anoxia and both displayed an enhanced CEF when compared with that measured in oxic conditions. As recast in Table 2 , the comparison of the three strains, ptox2 , stt7 and wild type, shows that: (i) CEF is similarly enhanced in the three strains under anoxic conditions suggesting that it is controlled by the intracellular reducing power, and that (ii) state transitions, although obviously not exclusive of the enhancement of CEF, are neither necessary nor sufficient to tune CEF. This contradicts previous studies that all supported a strong correlation between transition to State 2 and the enhancement of CEF in C. reinhardtii [8] , [12] , [45] . This contradiction may stem from the different observable used to measure CEF in these previous studies. They relied on the redox state of cytochrome f and not of P 700 as a probe of CEF, so that the transient acceptor side limitation undergone by PSI ( Fig. 5 ) that, to our knowledge, had not been reported at that time, likely escaped the attention of the authors. Thus, different light-induced redox states of cytochrome f between different strains might have been interpreted as reflecting changes in the reduction rate, that is, in CEF efficiency, whereas they likely reflected different degree of charge recombination within PSI and the consecutive changes in the light-induced oxidation rate of cytochrome f . CEF supercomplexes are formed independently of ST By demonstrating, at the molecular level, that some actors involved in LEF may be specifically recruited for CEF under State 2 conditions, the isolation of a PSI– b 6 f super-complex has brought considerable support to the model linking the efficiency of CEF to the structural reorganization associated with state transition [13] . This study, confirmed recently by Terashima et al . [33] , showed that this super-complex is more abundant in State 2 conditions than in State 1. Yet, it left open the question as to whether the association of LHCII to PSI is the structural determinant of CEF complex formation. We therefore compared the wild type, stt7 and ptox2 strains for their ability to form the super-complex, in oxic and anoxic conditions. For oxic conditions, ptox2 cells were simply kept well aerated in the dark to preserve, as detailed above, the association of mobile LHCII to PS I. To avoid the reduction of the plastoquinone pool that might result from the high cell concentration required for breakage in the French press, we subjected the culture to illumination in the presence of DCMU. The same treatment was applied to stt7 . After solubilization of wild-type thylakoid membranes with tridecyl-maltoside and separation on a sucrose density gradient, we found, in agreement with Iwaï et al . [13] , a green band of high molecular weight that was abundant in anoxic but undetectable in oxic conditions ( Fig. 6a ). The bulk of the LHCII was always found in the upper fractions, disconnected from both photosystems, as previously observed by Iwaï et al. [13] Western blot analysis ( Fig. 6b ) showed that the high-molecular weight band contained PS I, the b 6 f complex, FNR, PetO and PGRL1, all components already identified by Iwaï et al. [13] as part of the ‘CEF super-complex’. Importantly, this band was also observed in stt7 cells placed in anoxia, despite the lack of Stt7-dependent phosphorylation, and it was not present in oxic ptox2 cells, even though they were already in State 2, as evidenced by their phosphorylation pattern and low-temperature fluorescence emission spectrum ( Fig. 2 ). Actually, the results of membrane protein fractionation in the three strains were practically indistinguishable, as viewed both by the chlorophyll distribution and by western blot analysis. 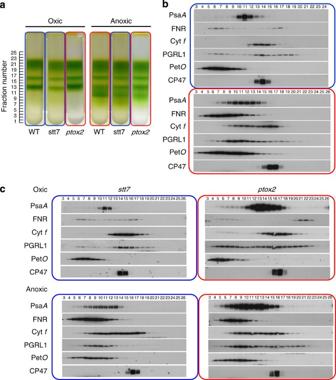Figure 6: Formation of CEF supercomplexes upon shift from oxic to anoxic conditions. Panelashows the sucrose density gradient in the wild type,stt7andptox2strain in oxic (left) and anoxic conditions (right). The blue frames indicate State 1, the red frames State 2. In all strains, a high-molecular weight green band was found in anoxic, but not in oxic conditions. Western blot analysis of the gradients (panelsbandc) showed that this high-molecular weight band (in fractions 8–12) contains PS I, theb6fcomplex, FNR, PetO, PGRL1 in good agreement with the study by Iwaiet al.13Fractions were loaded on an equal volume basis. Figure 6c shows the fractionation patterns of the mutants, and both display the same reorganization as the wild type, that is, the appearance in fractions 9–11 of PSI, cytochrome b 6 f and the other reported components of the CEF super-complex. Importantly, these proteins were never seen at that position in experiments performed with oxic cells, be they in State 1 (wild type, stt7 ) or in State 2 ( ptox2 ). Saliently, the amount of FNR retained in the membrane fraction increased dramatically in anoxic conditions in the three strains under study ( Fig. 6b and c ). In contrast to oxic conditions, it distributed only in high-molecular weight fractions after sucrose density centrifugation, with a pattern similar to that of PetO. Thus the redox state of some still unidentified molecular entities may tune the affinity of FNR for a membrane-bound protein complex that may contain PetO. As regards to this issue, we note that, in oxic conditions, part of PGRL1 was found in high-molecular weight fractions that contained FNR and PetO, but neither PSI nor b 6 f . With the qualification that co-distribution does not necessarily imply interactions, this observation suggests the existence of high-molecular weight complexes harboring at least these three proteins that could act as a pre-complex that eventually would be recruited to promote formation of a CEF super-complex. Figure 6: Formation of CEF supercomplexes upon shift from oxic to anoxic conditions. Panel a shows the sucrose density gradient in the wild type, stt7 and ptox2 strain in oxic (left) and anoxic conditions (right). The blue frames indicate State 1, the red frames State 2. In all strains, a high-molecular weight green band was found in anoxic, but not in oxic conditions. Western blot analysis of the gradients (panels b and c ) showed that this high-molecular weight band (in fractions 8–12) contains PS I, the b 6 f complex, FNR, PetO, PGRL1 in good agreement with the study by Iwai et al . [13] Fractions were loaded on an equal volume basis. Full size image The present results unambiguously show that the efficiency of CEF is not correlated with the phosphorylation and lateral migration of the mobile LHCII antenna toward PSI. The accumulation of reducing power and transition to State 2 do coincide in the wild type, with the result that the latter will contribute to the enhancement of CEF in light-limiting conditions, as discussed in the study by Cardol et al . [46] However, we clearly show here that cells switch from a low CEF to a high-CEF state in anoxia even in the absence of reorganization of their antenna, and that this switch most likely relies on a redox control. In addition, our results bring support to the notion that the regulation of CEF relies on the formation of supercomplexes that bring together within a single biochemical entity the actors involved in CEF. The mechanism by which the increase in reducing power promotes CEF and formation of these supercomplexes remains to be unraveled at the molecular level. We have ruled out here the involvement of the Stt7-dependent phosphorylation and antenna reorganization. Yet, the present data do not rule out the possible implication of other kinase(s) than Stt7, such as Stl1/STN8 [47] , [48] , [49] , [50] , when the redox conditions are such that CEF is enhanced. Saliently, by making the chloroplast-reducing power the main determinant of the enhancement of CEF, we provide a mechanistic model that likely applies to the entire green lineage including the vast majority of the cases known to date in which the redistribution of the LHCII occurring upon state transition involves a limited fraction of the antenna. Prominent among these are C3 plants in which CEF has been shown to be promoted in conditions where the pool of the PSI electron acceptors is over-reduced [51] , [52] , [53] . Strains and growth conditions In this study, we used the C. reinhardtii wild-type strain t222+ (hereafter wild type), derived from multiple backcrosses of the 137c strains [15] , the ‘stt7-9’ strain (hereafter stt7 (ref. 18 )) used in the study by Cardol et al . [46] , and the ptox2 mutant described in the study by Houille-Vernes et al . [15] Cells were grown to mid-log phase (3–5 × 10 6 cells per ml) in Tris acetate-phosphate medium (TAP) at 25 °C under cool fluorescent light (50 μmol photons m −2 s −1 ). Induction of State 1 and State 2 and isolation of thylakoid membranes Wild type and mutant cells were harvested by centrifugation (2,800 g , 5 min, 25 °C) and resuspended in a small volume of the initial growth medium. To induce State 1, cells were suspended at 5 × 10 7 cells per ml, wild type and stt7 were illuminated at 800 μE m −2 s −1 in the presence of 10 μM 3-(3,4-dichlorophenyl)-1,1-dimethylurea (DCMU) for 20 min. For State 2 in oxic conditions, ptox2 cells, resuspended at 5 × 10 7 cells per ml, were strongly agitated in the dark for 20 min. For anoxic treatment, cells were suspended at 2 × 10 8 cells per ml and incubated in the presence of 100 mM glucose, 2 mg per ml glucose oxidase from Aspergillus niger (Sigma-Aldrich, USA) and 50 units per ml catalase from A. niger (Sigma-Aldrich, USA) in the dark for 40 min. Thylakoid membranes were isolated as described in the study by Chua et al . [54] with modifications as in the study by Takahashi et al . [55] , except that broken cells were collected in a large volume of buffer containing 25 M Hepes-KOH pH 7.5, 5 mM MgCl 2 , 0.3 M Sucrose. For the preparation of membranes from anoxic samples, we added 100 mM glucose, 0.2 mg per ml glucose oxidase and 50 units per ml catalase from bovine liver (Sigma-Aldrich, USA) in all buffers. Samples were frozen in liquid nitrogen and stored at −80 °C. Sucrose density gradient ultracentrifugation Thylakoid membranes were thawed on ice and solubilized with 0.85% ( w / v ) n -Tridecyl-β- D -maltoside (TDM; Applichem, Germany) on ice for 20 min and subsequently loaded on sucrose density gradients (0.1–1.3 M sucrose, 5 mM Tricine-NaOH pH 8.0, 0.005% TDM) and centrifuged at 38,000 r.p.m. (SW41Ti; Beckman Coulter, USA) at 4 °C for 24 h. Fractions were collected from the bottom after piercing with a 22-G needle. The chlorophyll distribution along the gradient was assayed by the absorbance at 680 nm. SDS–PAGE and immunoblotting analysis Proteins from thylakoid membranes and fractions of sucrose density gradient centrifugation were solubilized with 2% SDS and 0.1 M dithiothreitol. Thylakoids were heated at 100 °C for 1 min, fractions at 80 °C for 5 min. SDS–PAGE was done according to the study by Laemmli [56] in Mini-Protean system (Bio-Rad, USA) or wide-mini cool slab (Bio Craft, Japan) apparatus. Immunoblotting was performed as described in the study by Takahashi et al . [55] Phosphorylation assay To detect phosphorylated proteins by immunoblotting, the cells were prepared as follows: wild type and mutant cells were harvested by centrifugation (2,800 g , 5 min, 25 °C) and resuspended in a small volume of their growth medium at 6 × 10 6 cells per ml. To induce State 1, cells were illuminated at 200 μE m −2 s −1 in the presence of 10 μM 3-(3,4-dichlorophenyl)-1,1-dimethylurea (DCMU) for 20 min. For anoxic treatment and to induce State 2, cells were incubated in the presence of 100 mM glucose, 2 mg per ml glucose oxidase from A. niger (Sigma-Aldrich, USA) and 50 units per ml catalase from A. niger (Sigma-Aldrich, USA) in the dark for 40 min. As a third condition, referred to as oxic (dark and agitation) conditions, cells were vigorously stirred in the dark for 20 min. The cell were resuspended in cold 5 mM Hepes buffer containing 10 mM EDTA and 10 mM NaF and were then collected by centrifugation. Collected cells were suspended into 0.1 M DTT and Na 2 CO 3 and frozen in liquid nitrogen. Total cellular proteins were solubilized in 2% SDS, heated at 100 °C for 1 min, separated on a 8 M urea 12–18% acrylamide gel [57] and transferred to a nitrocellulose membrane. Phosphoproteins were revealed with a phospho-threonine antibody (#9381, Cell signaling Technology, Inc., USA). The signals were detected by enhanced chemiluminescence (ECL, GE Healthcare). Spectrophotometric measurements Prior to spectrophotometric measurements, cells were grown in TAP medium to 3 × 10 6 cells per ml. They were centrifuged at 4,000 r.p.m. for 5 min at 20 °C, and the pellet was resuspended in HEPES 20 mM pH 7.2, 10% Ficoll to reach 6 × 10 6 cells per ml. The cells (5–10 ml) were then vigorously stirred in a 50 ml Erlenmeyer for 30 min in the dark, at 340 r.p.m. Strict anoxia was reached by addition of glucose oxidase (Type II, A. niger —2 mg ml −1 ), catalase (50 units per ml) and glucose (20 mM). Absorption changes were measured as described previously in the study by Alric et al . [32] with a JTS-10 spectrophotometer (Bio-Logic, Grenoble). The detecting and continuous lights were provided by LEDs and the saturating flash by a dye laser (640 nm) pumped by a the second harmonic of a Nd:Yag laser (Minilite II Continuum). The detection wavelength was selected using interferential filters: for measurement of electrochromic shift, 520 nm, 10 nm FWHM; for P 700 , 705 nm, 6 nm FWHM. Blue filters (BG-39, Schott) were used to cut off the excitation light. For P 700 , the absorption changes measured at 730 nm were subtracted to correct for unspecific contribution at 705 nm. DCMU (10 μM) was added just before measurement. Each measurement was made with a fresh sample to avoid any light-induced state transition. Assessment of the PSI antenna size To assess the PSI antenna size, we used the peak of the electrochromic shift (ECS) of carotenoid molecules borne by antenna proteins, caused by a light-induced change in the amplitude of the transmembrane electric field [58] . In green organisms like C. reinhardtii , the increase in absorption at 520 nm is proportional to the light-induced transmembrane electrical field and thus provides a direct measure of the number of charges that are transferred, upon illumination, from one side of the membrane to the other [59] . The slope of the light-induced absorption changes is thus proportional to the number of charges transferred per unit of time (see Fig. 3 ). In addition, the amplitude of the ECS measured after a single-turnover flash in the presence of DCMU provides an internal standard allowing calibration of the signal (one charge transferred per PSI). Based on this calibration, the y axis can be scaled and expressed in number of electron transferred per PSI (right y axis). When measured with respect to this thereby scaled axis, the slope of the absorption changes under continuous illumination gives rate at which ECS builds-up, directly in e − s −1 per PSI. This rate is not only proportional to the light intensity, but also to the PSI absorption cross section or, in short, its antenna size. It is noteworthy that, on this short time scale, the decay of the ECS through H+ conductance is negligible. Low-temperature fluorescence emission spectra Low-temperature emission spectra were measured using a laboratory built set-up. The samples, prepared as just described above, were placed in an aluminium sample holder that was plunged into liquid nitrogen. The fluorescence exciting light was provided by a LED (λ max 450 nm, LS-450, Ocean Optics) and shone onto the sample using a Y-shaped optical fiber. The other branch of this fiber was connected to a CCD spectrophometer (QE6500, sOcean Optics) to measure the emission spectrum. Cyclic electron flow Cyclic electron flow was estimated as in the study by Alric et al . [32] , in the presence of 10 μM DCMU to inhibit PS II activity. Under continuous illumination, at steady state, k ox [P 700 red ]= k red [P 700 ox ], where k ox stands for the oxidation rate of P 700 red and k red , the reduction rate of P 700 ox . Thus, CEF determination requires the knowledge of k ox [P 700 red ]. k ox , which is a convolution of the light intensity and the PSI antenna size, was assessed using the electrochromic shift as illustrated in Fig. 3 . [P 700 red ], the fraction of P 700 remaining reduced in the light was assessed as in the studies by Klughammer and Schreiber [35] and Baker et al . [60] . The electron flux sustained under these conditions is simply the product between k ox and P 700 red . Importantly, the flow rates measured were not kinetically limited by the light intensity, as increasing the light intensity yielded flow rates of similar values. How to cite this article: Takahashi, H. et al . Cyclic electron flow is redox-controlled, but independent of state transition. Nat. Commun. 4:1954 doi: 10.1038/ncomms2954 (2013).